Observation of detection-dependent multi-photon coherence times The coherence time constitutes one of the most critical parameters that determines whether or not interference is observed in an experiment. For photons, it is traditionally determined by the effective spectral bandwidth of the photon. Here we report on multi-photon interference experiments in which the multi-photon coherence time, defined by the width of the interference signal, depends on the number of interfering photons and on the measurement scheme chosen to detect the particles. A theoretical analysis reveals that all multi-photon interferences with more than two particles feature this dependence, which can be attributed to higher-order effects in the mutual indistinguishability of the particles. As a striking consequence, a single, well-defined many-particle quantum state can exhibit qualitatively different degrees of interference, depending on the chosen observable. Therefore, optimal sensitivity in many-particle quantum interferometry can only be achieved by choosing a suitable detection scheme. The coherence time is the timescale over which wave-like interference is observed for a particle-like object. In practice, it constitutes the critical parameter that determines whether or not quantum interference is observed in an experiment. It intimately characterizes quantum systems, such as, photons [1] , [2] , electrons [3] and molecules [4] . For photons, the traditional notion of coherence time is determined by the photon generation process and the bandwidth of spectral filtering [1] , [5] . Consider now the two-photon interference experiment first conducted by Shih and Alley [6] and Hong et al . [1] , where two single photons impinge on a 50:50 beam splitter (BS) via different input ports. When the photons are indistinguishable, that is, when they impinge within their coherence time, they always leave the BS in coalescence, due to the destructive interference of the amplitudes associated with two reflected and two transmitted photons. If these amplitudes become distinguishable, even in principle, interference is lost and the coalescence breaks up [7] , [8] . Distinguishability may originate, for instance, from different arrival times [1] , polarization states [9] , group velocity dispersion [10] and spectral distribution [5] of the two photons. In such experiments, the interference signal is observed in coincidence measurements between two single-photon detectors located at the output ports of the BS. When a single-photon detector is placed at each output port and temporal distinguishability is adjusted, the coincidence measurement exhibits the typical Hong–Ou–Mandel dip [1] . Consequently, for two single-photon detectors that are combined with a BS and thus function as a two-photon detector at one output port, a peak appears [2] . The peak and the dip in these two-photon signals have the same width and are directly related to the single-photon coherence time [1] , [2] , which is determined by the spectral properties of the photon [1] , [5] . At this stage, the single-photon coherence time seems to adequately characterize the shape of measurable multi-photon signals. By injecting a two-photon Fock-state [11] or a three-photon Fock-state [12] into each input mode of the aforementioned setup and by detecting all photons (four or six, respectively) at one output port of the BS, similar coincidence peaks have been observed. Defining the multi-photon coherence time as the width of the multi-photon signal, how do general multi-photon coherence times depend on the single-photon coherence time? More importantly, is the multi-photon coherence time always unambiguously determined by the single-photon coherence time? Here, we answer these questions experimentally and theoretically. We show in two- and four-photon interference experiments that the measured coherence time depends on the number of interfering photons and on the measurement scheme used to detect the particles. The unique two-photon coherence time that is determined by the single-photon coherence time turns out to be a rather accidental exception. In particular, an asymmetric four-photon detection scheme leads to a significant reduction of the observed coherence time. A theoretical study reveals that multi-photon signals depend on various powers of the indistinguishability (to be quantified in equation 1, below) of the interfering photons. As these different terms kick in as soon as more than two photons are brought to interference, our results imply that generic multi-photon coherence times depend on the number of interfering photons and on the chosen detection scheme, and, in general, that they are not simply determined by the single-photon coherence time. Experimental setup The experimental setup for observing such multi-photon coherence times is shown in Fig. 1 . Photon pairs are generated via spontaneous parametric down-conversion (SPDC), they are subsequently led to the input modes a and b of the BS. The temporal distinguishability of photons in a and b is controlled by adjusting the time delay τ of the photons in b . We observe two-photon interference (for single-photon Fock-states in a and b ) and four-photon interference (for two-photon Fock-states in a and b ) by twofold and fourfold coincidence detection, respectively. See Methods for Fock-state postselection. To investigate the questions posed above, we compare two different detection schemes: either all four detectors are placed at mode c only, which is used for the detection of (2,0) or (4,0) photons in modes c and d ( Fig. 1a ), or three detectors are placed in c and one in d , allowing (1,1)- and (3,1)-detection ( Fig. 1b ). 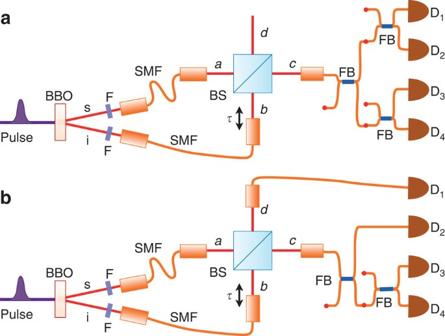Figure 1: Experimental setup. A frequency-doubled vertically polarized laser pulse with a pulse width of ~200 fs (central wavelength: 390 nm, average power: 120 mW) from a mode-locked Ti:Sa laser is focused onto a type-I β-barium-borate (BBO, thickness: 2 mm) crystal by a lens (not shown) with a focal length of 300 mm. Horizontally polarized signal (s) and idler (i) photons are generated via non-collinear frequency-degenerate spontaneous parametric down-conversion (SPDC) and filtered by a set of narrow bandpass filters (F). They are centred at 780 nm with FWHM of 4 nm. The signal and idler photons are then coupled into single-mode fibres (SMF) for cleaning up the spatial modes. The outputs of the SMFs are collimated and compensated for polarization rotation, induced by the propagation through the SMFs, with a set of half-wave and quarter-wave plates (not shown). The photons are then combined at a 50:50 beam splitter (BS). The temporal overlap of the photons at the BS is controlled by adjusting the arrival time delayτbetween the signal and the idler photons with a fibre collimator attached to a motorized stage located at the input modebof the BS. Photons are then detected at the output modes (candd) of the BS with single-photon detectors D1~D4(Perkin-Elmer SPCM-AQ4C) coupled to single-mode fibres and 50:50 fibre beam splitters (FB), the coincidence window is less than 8 ns. Different detector arrangements permit to detectmandnphotons at the output modescandd, respectively, denoted by (m,n)-detection. Detection of (2,0) and (4,0) can be observed inaand detection of (1,1) and (3,1) can be observed inb. Figure 1: Experimental setup. A frequency-doubled vertically polarized laser pulse with a pulse width of ~200 fs (central wavelength: 390 nm, average power: 120 mW) from a mode-locked Ti:Sa laser is focused onto a type-I β-barium-borate (BBO, thickness: 2 mm) crystal by a lens (not shown) with a focal length of 300 mm. Horizontally polarized signal (s) and idler (i) photons are generated via non-collinear frequency-degenerate spontaneous parametric down-conversion (SPDC) and filtered by a set of narrow bandpass filters (F). They are centred at 780 nm with FWHM of 4 nm. The signal and idler photons are then coupled into single-mode fibres (SMF) for cleaning up the spatial modes. The outputs of the SMFs are collimated and compensated for polarization rotation, induced by the propagation through the SMFs, with a set of half-wave and quarter-wave plates (not shown). The photons are then combined at a 50:50 beam splitter (BS). The temporal overlap of the photons at the BS is controlled by adjusting the arrival time delay τ between the signal and the idler photons with a fibre collimator attached to a motorized stage located at the input mode b of the BS. Photons are then detected at the output modes ( c and d ) of the BS with single-photon detectors D 1 ~D 4 (Perkin-Elmer SPCM-AQ4C) coupled to single-mode fibres and 50:50 fibre beam splitters (FB), the coincidence window is less than 8 ns. Different detector arrangements permit to detect m and n photons at the output modes c and d , respectively, denoted by ( m , n )-detection. Detection of (2,0) and (4,0) can be observed in a and detection of (1,1) and (3,1) can be observed in b . Full size image Experimental results First, two-photon interference of single-photon Fock-states in input modes a and b is observed [1] , [2] . The detection of two photons at one output mode, (2,0)-detection, is conducted by twofold coincidence detection by D 1 and D 3 in the configuration shown in Fig. 1a . The coincidence counts exhibit a peak with a width of σ (2,0) =373±7 fs (we always refer to the full width at half maximum, FWHM), which is a manifestation of the two-photon coalescence effect, see Fig. 2a (ref. 2 ). The enhancement factor, that is, the ratio of the counts at τ =0 and τ =∞, amounts to 1.93±0.02. On the other hand, single-photon detection at both output ports, that is, (1,1)-detection, is conducted by twofold coincidence detection by D 1 and D 2 in the configuration of Fig. 1b . We observe a typical Hong–Ou–Mandel dip [1] , [6] , shown in Fig. 2b , with a width of σ (1,1) =379±5 fs, which is very close to σ (2,0) . As we shall show later in the analysis, this equality perfectly matches the theoretical expectation. 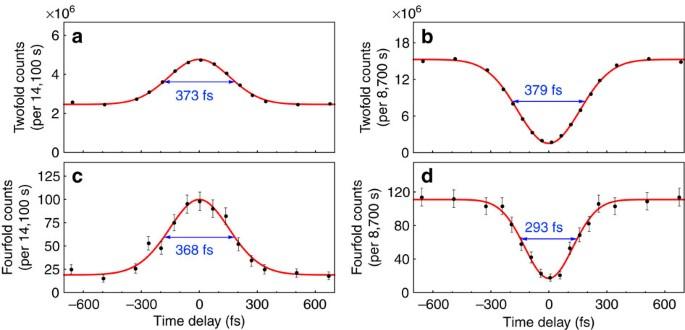Figure 2: Two- and four-photon interference observed under different detection schemes. The detection schemes used are (2,0)-detection ina, (1,1)-detection inb, (4,0)-detection incand (3,1)-detection ind. Solid circles are experimental data, and solid lines are the best fits to the data using the fitting functions from our theoretical model, see equation 2. Error bars represent one s.d. from Poissonian counting statistics. The (3,1)-detection signal exhibits a significant width reduction with respect to the (4,0)-detection signal. Figure 2: Two- and four-photon interference observed under different detection schemes. The detection schemes used are (2,0)-detection in a , (1,1)-detection in b , (4,0)-detection in c and (3,1)-detection in d . Solid circles are experimental data, and solid lines are the best fits to the data using the fitting functions from our theoretical model, see equation 2. Error bars represent one s.d. from Poissonian counting statistics. The (3,1)-detection signal exhibits a significant width reduction with respect to the (4,0)-detection signal. Full size image A qualitatively different picture is encountered for four-photon interference. As described above, a two-photon Fock-state is injected into each input mode ( a and b ), and the four photons are detected under two different schemes: (4,0)-detection ( Fig. 1a ) and (3,1)-detection ( Fig. 1b ). The (4,0)-signal presented in Fig. 2c exhibits a peak with a width of σ (4,0) =368±27 fs and an enhancement factor of 5.3±0.8, in agreement with the value 6 expected for four-photon bunching [11] . The width is comparable to the two-photon width, with σ (4,0) / σ (1,1) =0.97±0.07. The (3,1)-signal, on the other hand, exhibits a dip, as shown in Fig. 2 d , as the four-photon path amplitudes that lead to (3,1)-events interfere destructively [13] . The width of the (3,1)-detection signal amounts to σ (3,1) =293±13 fs, the ratio of the widths is σ (3,1) / σ (1,1) =0.77±0.04. Clearly, the dip in the (3,1)-signal is significantly narrower than the peak in the (4,0)-signal, whereas the widths of the two-photon interference signals coincide, regardless of the detection scheme. We stress that these different widths result only from the choice of different detection events, as any other conditions such as spectral filtering are the same. The width of multi-photon interference signals is usually interpreted as the coherence time of the interfering photons, but our above observations show that a four-photon state cannot be assigned a unique coherence time. In stark contrast to two-photon quantum interference, the choice of the observed detection event becomes relevant for the shape of the observed signal, as our subsequent analysis explains. Theoretical analysis For a quantitative understanding of the observed behaviour, we operationally define the indistinguishability between two photons with time delay τ via the overlap of their amplitudes, where is a creation operator for a photon arriving at the BS centred at time t . Two photons are fully indistinguishable for =1 and fully distinguishable for =0; for most quantum states, such as the frequently encountered Gaussian states (see Methods), these cases are attained for τ =0 and τ =∞, respectively. When an ( N /2)-photon Fock-state enters at each input mode of a BS, the state of the delayed photons in mode b can be decomposed into a superposition of N /2+1 states, each term consisting of d (=0,1,…, N /2) distinguishable and N /2− d indistinguishable photons with respect to any photon in mode a (refs 14 , 15 ). Each term that describes d distinguishable photons at mode b , together with the ( N /2)-photon Fock-state in mode a , is denominated of d -distinguishability type. The weight of each type is a function of up to a power of N /2. As a result, the overall detection probability for the ( N − m , m ) outcome is a polynomial in with a maximal power N /2, as explained in more detail in the Methods section. With equation 2 at hand, we can understand the observed two-photon and four-photon interference signals: the different detection schemes in Fig. 1 result in distinct multi-particle interference paths [15] , and, consequently, result in distinct coefficients , as shown in Table 1 . As a consequence, the resulting signals differ. Table 1 Coefficient of k -th power of indistinguishability. Full size table To model the observations, we need to account for the Gaussian frequency distribution of the photons in our experimental setup. We denote the resulting width of the indistinguishability (equation 1) by Δ τ , the width of higher orders is then reduced by a factor of (see Methods). For two-photon interference, only the linear contribution contributes to the detection probabilities ( Table 1 ); thus, both P (2;2,0) ( τ ) and P (2;1,1) ( τ ) exhibit the same width, and a unique coherence time can be assigned to the two-photon state. When four photons interfere, quadratic terms proportional to emerge in the detection probabilities ( Table 1 ). For P (4;4,0) ( τ ), both and contribute, but the linear term has a larger prefactor, such that it dominates the overall behaviour. Consequently, the signal width is only slightly reduced with respect to two-photon interference, it amounts to ~0.93Δ τ , in good agreement with the measured value σ (4,0) / σ (1,1) =0.97±0.07. On the other hand, for P (4;3,1) ( τ ) only the quadratic term contributes and the resulting width amounts to , which is significantly narrower and coincides well with the experimentally observed value σ (3,1) / σ (1,1) =0.77±0.04. In other words, the second-order power of the indistinguishability determines the width of the multi-photon signal and induces the hierarchy σ (3,1) < σ (4,0) < σ (1,1) = σ (2,0) =Δ τ . When the number of interfering photons is increased further, higher orders of the indistinguishability become relevant. In N -photon interference, up to N /2-th order effects of the indistinguishability emerge in equation 2, and each k -th power of the indistinguishability leads to a signal with a particular width. The coefficients , which are determined by the chosen detection scheme [15] , then regulate which power of the indistinguishability dominates the sum and determine the observed multi-photon coherence time. Therefore, no unique coherence time can be assigned to a multi-photon state. The dependence on the detection scheme is an innate property of multi-photon states [16] , which takes place irrespective of the specific shape of . In particular, the multi-photon coherence time associated with the detection of ( N ,0) decreases with increasing number of photons N . For the Gaussian frequency distribution, the ratio σ ( N ,0) / σ (1,1) converges to the asymptotic value (see Methods), shown as a red dashed line in Fig. 3 . On the other hand, coherence times related to the detection of the ( N − m , m ≠0)-signal typically increase with the number of photons N . As an example, see the widths of the ( N /2, N /2)-signal and of the ( N /2−2, N /2+2)-signal for odd N /2, and the ( N /2+1, N /2−1)-signal for even N /2 shown in Fig. 3 . The increase of the signal width can be understood from the strong interference that is exhibited by a Fock-state interfering with a single photon [17] : the ( N /2–1)-distinguishability type describes such a state with exactly one indistinguishable photon, which naturally features strong interference. With increasing particle number N , the ( N /2−1)-distinguishability type becomes not only broader, but also more influential. In general, the widths of ( N ,0) and ( N − m , m ≠0)-signals exhibit opposite tendencies for increasing number of photons N , and the dependence of the observed multi-photon coherence times on the chosen event becomes more and more dramatic as more photons interfere. 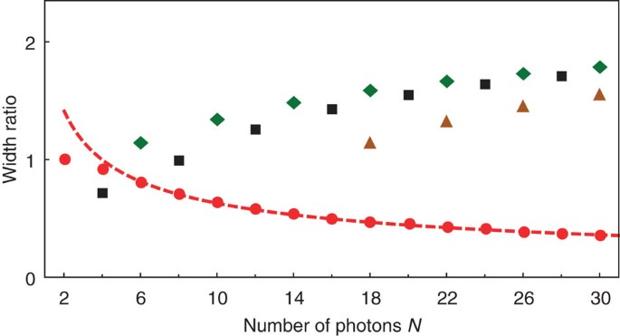Figure 3: Relative multi-photon coherence times. Relative coherence times as a function of the number of photons, quantified by width ratiosσ(N−m,m)/σ(1,1), are shown for photons with Gaussian frequency distribution (equation 9). Circles (red), diamonds (green), squares (black) and triangles (brown) represent the width ratios for the detection of (N,0), (N/2,N/2), (N/2+1,N/2−1) and (N/2+2,N/2−2), respectively. The dashed (red) line is the asymptotic expressionfor the width ratio of the (N,0)-signal. Figure 3: Relative multi-photon coherence times. Relative coherence times as a function of the number of photons, quantified by width ratios σ ( N − m , m ) / σ (1,1) , are shown for photons with Gaussian frequency distribution (equation 9). Circles (red), diamonds (green), squares (black) and triangles (brown) represent the width ratios for the detection of ( N ,0), ( N /2, N /2), ( N /2+1, N /2−1) and ( N /2+2, N /2−2), respectively. The dashed (red) line is the asymptotic expression for the width ratio of the ( N ,0)-signal. Full size image In conclusion, the possibility to measure the single-photon coherence time via the width of the two-photon interference signal turns out to be rather accidental. We have shown in experiment and in theory that the multi-photon coherence time, as defined by the width of the observed multi-photon signal, is not unique. Instead, it depends on the number of interfering particles and on the very way the photons are detected. Thus, to a great extent, the strength of quantum multi-particle interference depends on the chosen observable. Fock-states postselection The quantum state of the photon pairs generated via spontaneous parametric down-conversion is proportional to , where is the single pair generation probability. Each component contains a Fock-state with an equal number of photons at the modes a and b . As =0.028 in the experiment, twofold and fourfold coincidences are attributed with high certainty to the respective states |1,1 a , b and |2,2 a , b at the input modes of the BS. Wave-function decomposition The quantum state of N /2 photons in mode a and N /2 photons in the delayed mode b is given as where denotes the creation operator for a photon in mode a ( b ). The creation operator for a delayed photon in b can be written as a superposition of one indistinguishable (that is, parallel) and one distinguishable (that is, orthogonal) component with respect to a photon in a : where is the indistinguishability given in equation 1 and is the creation operator that takes into account the part of the wave-function in b that is orthogonal to the wave-function of a photon in a . In other words, each photon in b is indistinguishable with respect to the photons in a with probability . By substitution of equation 4, the multi-photon state in equation 3 becomes where we can identify N /2+1 different d- distinguishability types, that is, terms with a fixed number d of distinguishable and N /2− d of indistinguishable photons in b with respect to the photons in a , together with the N /2 photons in a (refs 14 , 15 ). For each type, N /2− d photons in b interfere with the photons in a , whereas the remaining d photons do not. The weight of the d -distinguishability type is a polynomial in , given as which can be deduced from equation 5. Overall detection probability As each d -distinguishability type is orthogonal to all other distinguishability types, the overall detection probability for the outcome ( N − m , m ) is the mean of the detection probabilities associated with each d -distinguishability type (refs 13 , 18 , 19 ), weighted by : As contains up to a power of N /2, the overall detection probability is a polynomial in with a maximal power of N /2, which can be expressed by equation 2. In particular, the probability for ( N ,0)-detection results in a k -th order coefficient in equation 2 corresponding to the square of a binomial coefficient, such that the most important contribution is given by , which quickly becomes dominant as N increases. As a result, the width of the ( N ,0)-signal converges to the width of the N /4-th order of the indistinguishability, in the limit of large N . Photons with Gaussian frequency distribution A photonic creation operator with Gaussian frequency distribution is given by where t is the central arrival time of the photon at the BS and is the creation operator for a photon of frequency ω ; the central frequency is ω 0 and the bandwidth is Δ ω . In this case, the indistinguishability (equation 1) becomes , it is characterized by a FWHM of . The k -th power of the indistinguishability, , has a reduced FWHM of . How to cite this article: Ra, Y.-S. et al . Observation of detection-dependent multi-photon coherence times. Nat. Commun. 4:2451 doi: 10.1038/ncomms3451 (2013).